An ancestral NB-LRR with duplicated 3′UTRs confers stripe rust resistance in wheat and barley Wheat stripe rust, caused by Puccinia striiformis f. sp. tritici ( Pst ), is a global threat to wheat production. Aegilops tauschii , one of the wheat progenitors, carries the YrAS2388 locus for resistance to Pst on chromosome 4DS. We reveal that YrAS2388 encodes a typical nucleotide oligomerization domain-like receptor (NLR). The Pst -resistant allele YrAS2388R has duplicated 3’ untranslated regions and is characterized by alternative splicing in the nucleotide-binding domain. Mutation of the YrAS2388R allele disrupts its resistance to Pst in synthetic hexaploid wheat; transgenic plants with YrAS2388R show resistance to eleven Pst races in common wheat and one race of P . striiformis f. sp. hordei in barley. The YrAS2388R allele occurs only in Ae. tauschii and the Ae. tauschii -derived synthetic wheat; it is absent in 100% ( n = 461) of common wheat lines tested. The cloning of YrAS2388R will facilitate breeding for stripe rust resistance in wheat and other Triticeae species. Wheat ( Triticum spp.) is the largest acreage crop in the world. With an approximate 220 million hectares and 760 million tons in 2018, wheat was ranked second in global production after maize [1] . As a staple food crop, wheat provides about 20% of global calories for human consumption [2] . Because the world population is projected to increase by nearly two billion people within the next three decades [3] , the increasing human population worldwide will place an even greater demand for wheat production globally. Wheat stripe rust (or yellow rust; abbreviated as Yr), caused by Puccinia striiformis f. sp. tritici ( Pst ), is a serious fungal disease that poses a huge threat to wheat production in regions with cool and moist weather conditions [4] , including major wheat-producing countries, such as Australia, Canada, China, France, India, the United States, and many others [5] , [6] . Planting wheat cultivars with adequate levels of resistance is the most practical and sustainable method to control stripe rust. Host resistance of wheat against Pst is normally classified as either all-stage resistance (ASR) or adult-plant resistance (APR). Whereas ASR is effective starting at the seedling stage through the late stages of plant growth, APR is mainly effective at the late stages of plant growth [7] . In wheat, ASR confers high levels of resistance to specific Pst races, but the underlying genes, such as Yr9 [8] and Yr17 [9] , are often circumvented by the emergence of new virulent races. In contrast, APR typically provides a partial level of resistance, but is more durable and is effective against all or a wider spectrum of Pst races than ASR. High-temperature adult-plant (HTAP) resistance is a major type of APR; HTAP typically provides durable and non-race-specific resistance to Pst [10] . Incorporating multiple ASR and HTAP genes appears to be an excellent strategy for maintaining sustainable resistance to wheat stripe rust [10] . Over 80 wheat stripe rust resistance ( R ) genes ( Yr1–Yr81 ) have been permanently named [11] . Of the seven genes cloned so far, Yr5 , Yr7 and YrSP , a gene cluster, encodes nucleotide-binding (NB) and leucine-rich repeat (LRR) proteins [12] ; Yr15 has two kinase-like domains [13] ; Yr36 has a kinase domain and a lipid binding domain [14] ; Lr34/Yr18 encodes a putative ABC transporter [15] ; and Lr67/Yr46 encodes a predicted hexose transporter [16] . While the Yr5/Yr7/YrSP cluster and Yr15 confer ASR resistance to wheat stripe rust, Yr18 , Yr36 , and Yr46 confer APR or HTAP resistance. Of the three cloned APR genes, only the Yr18 gene has been widely used in wheat cultivars [17] ; however, Yr18 alone does not confer adequate resistance under high disease pressures. Yr7 and YrSP confer high levels of resistance, but Pst races virulent to Yr7 are common globally and those virulent to YrSP occur in some countries [18] . Yr5 and Yr15 confer high levels of resistance to a wide range of Pst races [12] , [19] , but the increasing adoption of them in wheat cultivars may cause the emergence of virulent races. Characterization of additional R genes is essential in order to assemble effective resistance to constantly changing populations of Pst . Aegilops tauschii Coss. (2 n = 2 × = 14, DD) is the D genome progenitor of common wheat [20] , [21] . The diverse Ae. tauschii D genome offers a valuable gene pool for stripe rust resistance [20] , [22] . To date, several stripe rust resistance genes have been mapped in Ae. tauschii , including YrAS2388 [23] and Yr28 [24] on 4DS [22] , [25] , and YrY201 [26] on 7DL. Synthetic hexaploid wheat (SHW) lines, which contain a diversity of Ae. tauschii accessions [27] , are potential breeding stocks. However, many biotic and abiotic resistance genes are suppressed in the hexaploid background [28] . To prevent a linkage drag of undesirable traits and resistance suppression, it is best to identify R genes and use them precisely in gene pyramids. In this study, we have cloned the stripe rust resistance gene YrAS2388 from Ae. tauschii . Additionally, we have demonstrated that this gene can express effectively in hexaploid wheat and barley. Deployment of YrAS2388R in wheat cultivars together with other effective genes should sustainably protect wheat production from the devastating disease wheat stripe rust. YrAS2388R confers resistance to wheat stripe rust Aegilops tauschii CIae9, PI511383 and PI511384 (all from the subspecies (subsp.) strangulata ) possess YrAS2388R [22] . 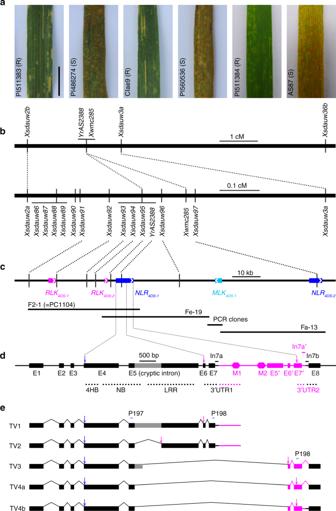Fig. 1 Map-based cloning of theYrAS2388gene.aAdult plant responses (R = resistant; S = susceptible) of parental lines to natural spores in the field. Scale bar = 1 cm.bGenetic maps are based on popC-1 (upper) and popA-2 (lower).cPhysical maps are based on three fosmid clones: F2-1 (= PC1104), Fe-19 and Fa-13, which contain five genes (colored rectangles; arrows pointing to 3′ ends) that encode for two 4-helix bundle-nucleotide binding-leucine rich repeat (NLRs), a malectin-like kinase (MLK), and two receptor-like kinases (RLKs). A 3.9-kb physical gap between Fe-19 and Fa-13 was closed by sequencing PCR clones.dGenomic structure ofNLR4DS-1in PI511383. The conserved domains and the duplicated 3′UTRs are labelled; their approximate genomic locations are highlighted with dotted lines. The 3′UTR duplication was caused by a 2668-bp insertion (magenta region), which has three regions (with a prime symbol) similar to exons 5, 6, and 7. Introns 7a and 7b, and exon 8 are the original components of the ancestral 3′UTR, but the 2668-bp insertion disrupted the ancestral 3′UTR and then formed two 3′UTRs, each containing both ancestral (black dots) and inserted (magenta dots) segments. The cryptic intron in exon 5 is highlighted by a gray box. Introns 7a, 7a′, and 7b have a size bar below their names.eTranscript variants ofNLR4DS-1in accession PI511383. Cloning and sequencing of theNLR4DS-1cDNA clones identified five transcript variants, designated TV1 to TV4b, ofNLR4DS-1in accession PI511383. Grey boxes indicate portions of the retained intron in mature messenger RNA. Rectangles and straight lines indicate regions present in mRNA; the caret-shaped lines represent regions that are absent in mRNA. Part of the cryptic intron in exon 5 is retained in TV3. TV4a and TV4b encode an identical protein, called TV4. P197 and P198 are primers that detect all five splicing variants in one PCR. Abbreviations include exon (E), four-helical bundle (4HB), intron (In), leucine-rich repeat (LRR), two miniature inverted-repeat transposable elements (M1 and M2), nucleotide-binding (NB), and start (downwards arrows in blue) and stop (downwards arrows in magenta) codons. Source data of Fig.1aare provided as a Source Data file At the two-leaf seedling (juvenile) stage, CIae9, PI511383, and/or PI511384 were resistant with infection types (IT) between 1 and 5 to nine Pst races (PSTv-3, PSTv-4, PSTv-11, PSTv-18, PSTv-37, PSTv-41, PSTv-51, PSTv-52, and PSTv-172), under low temperature (LT) and/or high temperature (HT) regimes (Table 1 ). These races are virulent on a wide range of wheat germplasm (Supplementary Data 1 ). CIae9, PI511383 and PI511384 have shown Pst resistance (IT scores = 1–3; Fig. 1a ) under natural infections in the Sichuan basin in China since 1995. In contrast, Ae. tauschii AS87, PI486274 and PI560536 (all subsp. tauschii accessions) do not have the YrAS2388R gene [22] , and were always susceptible under either natural infections or controlled inoculation (IT scores = 7–9; Fig. 1a , Table 1 ). Table 1 Seedling responses of selected lines to Puccinia striiformis f. sp. tritici Full size table Fig. 1 Map-based cloning of the YrAS2388 gene. a Adult plant responses (R = resistant; S = susceptible) of parental lines to natural spores in the field. Scale bar = 1 cm. b Genetic maps are based on popC-1 (upper) and popA-2 (lower). c Physical maps are based on three fosmid clones: F2-1 (= PC1104), Fe-19 and Fa-13, which contain five genes (colored rectangles; arrows pointing to 3′ ends) that encode for two 4-helix bundle-nucleotide binding-leucine rich repeat (NLRs), a malectin-like kinase (MLK), and two receptor-like kinases (RLKs). A 3.9-kb physical gap between Fe-19 and Fa-13 was closed by sequencing PCR clones. d Genomic structure of NLR 4DS-1 in PI511383. The conserved domains and the duplicated 3′UTRs are labelled; their approximate genomic locations are highlighted with dotted lines. The 3′UTR duplication was caused by a 2668-bp insertion (magenta region), which has three regions (with a prime symbol) similar to exons 5, 6, and 7. Introns 7a and 7b, and exon 8 are the original components of the ancestral 3′UTR, but the 2668-bp insertion disrupted the ancestral 3′UTR and then formed two 3′UTRs, each containing both ancestral (black dots) and inserted (magenta dots) segments. The cryptic intron in exon 5 is highlighted by a gray box. Introns 7a, 7a′, and 7b have a size bar below their names. e Transcript variants of NLR 4DS-1 in accession PI511383. Cloning and sequencing of the NLR 4DS-1 cDNA clones identified five transcript variants, designated TV1 to TV4b, of NLR 4DS-1 in accession PI511383. Grey boxes indicate portions of the retained intron in mature messenger RNA. Rectangles and straight lines indicate regions present in mRNA; the caret-shaped lines represent regions that are absent in mRNA. Part of the cryptic intron in exon 5 is retained in TV3. TV4a and TV4b encode an identical protein, called TV4. P197 and P198 are primers that detect all five splicing variants in one PCR. Abbreviations include exon (E), four-helical bundle (4HB), intron (In), leucine-rich repeat (LRR), two miniature inverted-repeat transposable elements (M1 and M2), nucleotide-binding (NB), and start (downwards arrows in blue) and stop (downwards arrows in magenta) codons. Source data of Fig. 1a are provided as a Source Data file Full size image Previously, we hypothesized that YrAS2388 and Yr28 are the same gene [22] . AvSYr28NIL and AvS are near-isogenic lines (NILs) for the Yr28 gene. During a Pst test with PSTv-3, PSTv-11, PSTv-41, and PSTv-172, AvS was susceptible to all races under both LT and HT, but AvSYr28NIL was highly resistant to PSTv-3, PSTv-11, and PSTv-172 (Table 1 ). We additionally tested two synthetic hexaploid wheat (SHW) lines, SW3 and SW58, that were derived from the durum wheat Langdon but have different D-genome donors: the Pst -resistant CIae9 and the Pst -susceptible AL8/78, respectively. Despite a dominant YrAS2388R gene in CIae9, SW3 was highly susceptible to PSTv-4, PSTv-18, PSTv-37 and PSTv-52 (Table 1 ), which was comparable to SW58 under LT. Thus, YrAS2388R can be suppressed when it is introgressed into certain hexaploid wheat genotypes. YrAS2388R was delimited to a 50-kb region in PI511383 CIae9, PI511383, PI511384 and eleven other accessions were found to have the YrAS2388R gene or allelic genes on 4DS [22] . We previously developed three F 2 populations: popA (PI511383/PI486274), popB (CIae9/PI560536) and popC (PI511384/AS87). The YrAS2388R -based Pst responses are inherited as a Mendelian trait in all three F 2 populations [22] . Here, among 1910 F 2 plants of popC-2 (PI511384/AS87), 1,432 were resistant and 478 were susceptible in Wenjiang, Sichuan, China, which fits single dominant gene inheritance (Chi-Square goodness of fit test, χ 2 3:1 = 0.001, P = 0.98). Using the wheat 10k iSelect array [29] , we genotyped CIae9, PI486274, PI511383, PI560536, and 17 Pst -susceptible F 2 plants (10 from popA and 7 from popB) for bulked segregant analysis (BSA) of the Pst -susceptible allele of YrAS2388 ( YrAS2388S ). Among 3276 applicable single nucleotide polymorphisms (SNPs), we selected 20 SNPs that were mostly associated with a Pst -susceptible phenotype; eight of them, including AT4D3406, AT4D3410, AT4D3411, AT4D3412, AT4D3413, AT4D3417, AT4D3418, and AT4D3419 (Supplementary Table 1 ), were in the 4DS distal region [29] . Based on specific genotypes per marker per plant, YrAS2388S was mapped distal to the AT4D3406 region (Supplementary Table 1 ). The AT4D3406 region (Supplementary Fig. 1a ) was initially targeted to map the YrAS2388 gene in popA and popC. Using the F 2 and F 3 data, we mapped YrAS2388 to the same region in popA-1 and popC-1 (Supplementary Fig. 1b, c ). 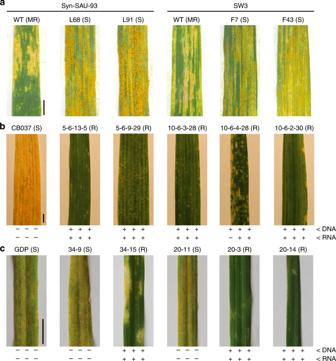Fig. 2 TheYrAS2388locus confers stripe rust resistance in wheat and barley.aSyn-SAU-93 and SW3 are two synthetic hexaploid wheat (SHW) lines that express theYrAS2388Rgene. WT is the resistant wild-type control with necrotic lesions. L68 (G117D), L91 (V267I), F7 (S394N) and F43 (V482I) are susceptible mutants with sporulatingPst. Plant responses (MR = moderate resistance; R = resistant; S = susceptible) toPstare indicated in parentheses.bThe susceptible hexaploid wheat CB037 was transformed with the intact PC1104 (= F2-1). Transgenic T3wheat (all from the No. 5 and 10 T2subfamilies) was challenged with PSTv-239 at the adult plant stage. Under each picture, PCR results as positive (plus signs) or negative (minus signs) for DNA amplification (upper) and RNA expression (lower) of the three target genes:RLK4DS-1(left),RLK4DS-2(middle) andNLR4DS-1(right). RT-PCR is illustrated in Supplementary Fig.4.cThe susceptible barley Golden Promise (GDP) was transformed with the intact PC1104 ( = F2-1). Transgenic T1barley seedlings were inoculated with race PSH-72 ofPuccinia striiformisf. sp.hordei(Psh). Scale bar = 1 cm. Source data are provided as a Source Data file In popC-1, YrAS2388 is between Xsdauw2b (= AT4D3403) and Xsdauw3a (= AT4D3405) (Supplementary Table 2 ), an approximate 2.4-cM interval (Supplementary Fig. 1c ). To assure that we defined the correct region, we targeted a large interval, Xsdauw2a (= AT4D3403) -Xsdauw36a (= AT4D3410), for screening recombinants in popA-2. Additional markers were designed from the linkage map [29] and genome sequence [30] of Ae. tauschii . First, we retrieved the AT4D3403, AT4D3404 and AT4D3405 corresponding genomic sequence [29] , prioritized the low-copy number regions, created nine PCR markers ( Xsdauw86 to Xsdauw91 , Xsdauw93 , Xsdauw95 and Xsdauw97 ) among six parental lines, and placed YrAS2388 between Xsdauw91 and Xsdauw97 (Supplementary Fig. 1d ). Second, we constructed a fosmid genomic library from the Pst -resistant genotype PI511383. Xsdauw92 , Xsdauw94 and Xsdauw96 were then developed using the fosmid clones of the YrAS2388 region. After analyzing 4205 popA F 3 plants, which were from 11 F 2 plants heterozygous in the Xsdauw2a-Xsdauw36a region, we precisely mapped YrAS2388 between Xsdauw92 and Xsdauw96 , about a 0.13-cM interval, and added to the YrAS2388 interval with three completely linked markers ( Xsdauw93 - Xsdauw95 ) (Fig. 1b , Supplementary Fig. 1d , Supplementary Table 2 ). The fosmid genomic library of PI511383 has approximately one million clones and represents an eight-fold coverage of the Ae. tauschii genome (≈ 4.3 Gb [30] ). Twenty fosmid clones were identified in the YrAS2388 region. In the physical map (Fig. 1c , Supplementary Fig. 2 ), Xsdauw91 and Xsdauw96 , which delimited the YrAS2388 gene, were anchored to the two overlapping fosmids, F2-1 and Fe-19. After sequencing F2-1 and Fe-19, we primarily analyzed the Xsdauw91-Xsdauw96 region (ca. 50 kb). RNA sequencing (RNA-seq) in PI511383 revealed three active genes in the Xsdauw91-Xsdauw96 interval, including two receptor-like kinase genes [31] ( RLK 4DS-1 and RLK 4DS-2 ), and a classic R gene, NLR 4DS-1 . Both RLK 4DS-1 and RLK 4DS-2 are wall-associated receptor kinases. RLK 4DS-1 has an N-terminal galacturonan-binding and a C-terminal serine/threonine kinase (STK) domain, whereas RLK 4DS-2 has only the STK domain. NLR 4DS-1 has a classic four-helix bundle (4HB) that was previously classified as a coiled-coil, a NB domain and a LRR domain with 12 or more leucine-rich repeats. All three genes are highly conserved among the Ae. tauschii accessions tested and the collinearity of the YrAS2388 region is conserved between Ae. tauschii and common wheat (Supplementary Fig. 2 ). Transcription of RLK 4DS-1 , RLK 4DS-2 and NLR 4DS-1 was confirmed by reverse-transcription PCR (RT-PCR) (Supplementary Fig. 3a, b ). Genome sequence analysis, RNA-seq and RT-PCR further revealed that the NLR 4DS-1 gene in PI511383 contains a 2668-bp insertion, which resulted in duplicated 3′ untranslated regions (3′UTR1 and 3′UTR2) and five transcript variants (Fig. 1d, e ). However, the NLR 4DS-1 gene in AL8/78 lacks the 2668-bp insertion and has only one transcript product. The closest distal marker, Xsdauw92 , placed RLK 4DS-1 outside of the YrAS2388 interval. Consequently, NLR 4DS-1 and RLK 4DS-2 became the most likely candidates for YrAS2388 . Both genes were expressed in the Pst -resistant parents (CIae9, PI511383 and PI511384) and in two Pst -susceptible genotypes (AL8/78 and AS87), but were inactive in two Pst -susceptible parents (PI486274 and PI560536) (Supplementary Fig. 3a, b ). In a comparison of NLR 4DS-1 in the Pst -resistant (CIae9, PI511383 and PI511384) and the Pst -susceptible (AS87 and AL8/78) genotypes, the cDNA and protein sequences are only 94% and 91% identical, respectively (Supplementary Data 2 ). The Pst -susceptible genotypes (AL8/78 and AS87) had a premature stop codon in RLK 4DS - 2 , which was absent in the Pst -resistant parents (CIae9, PI511383 and PI511384). Thus, both NLR 4DS-1 and RLK 4DS-2 remained as candidates for the YrAS2388 gene. Haplotype markers indicated that NLR 4DS-1 is YrAS2388 To help identify the correct gene, we genotyped 159 Ae. tauschii accessions using five markers for NLR 4DS-1 (HTM3a to HTM3e, or collectively called HTM3S), one for RLK 4DS-1 (HTM1a) and one for RLK 4DS-2 (HTM2a) (Supplementary Tables 2 and 3 , Supplementary Data 3 ). The R -type allele (e.g. “A” in PI511383) of NLR 4DS-1 was completely associated with Pst resistance in resistant haplotypes R1 to R3 (Supplementary Data 3 ). All non-A scores of the NLR 4DS-1 markers were associated with Pst susceptibility. The coding region (ATG to 3′UTR2; Fig. 1d ) of NLR 4DS-1 is identical amongst eight Pst -resistant Ae. tauschii accessions, including AS2386, AS2387, AS2399, AS2402, CIae9, PI349037, PI511383, and PI511384. In contrast, in RLK 4DS-1 and RLK 4DS-2 , the R -type allele (e.g. “A” in PI511383) was present in the Pst -susceptible genotypes (S1-S3 and S5), indicating that both genes do not confer Pst resistance. Similarly, the absence of RLK 4DS-1 and/or RLK 4DS-2 in the R2 and R3 haplotypes suggested that neither gene is essential for Pst resistance. Thus, NLR 4DS-1 is the only candidate for YrAS2388R . Pst -susceptible SHW mutants have more mutations in NLR 4DS-1 Synthetic hexaploid wheat (SHW) SW3 [32] and Syn-SAU-93 [33] acquire the YrAS2388R gene from their D-genome donor; both SW3 and Syn-SAU-93 displayed moderate Pst resistance (IT scores = 3–5; Fig. 2a ) in Sichuan, China. Using ethyl methanesulfonate (EMS), we generated 1132 M 2 families of SW3 and 613 M 2 families of Syn-SAU-93. Under field conditions, we identified 103 Pst -susceptible plants (IT scores = 7–9; Fig. 2a , Supplementary Data 4 ). For the NLR 4DS-1 , RLK 4DS-1 , and RLK 4DS-2 genes, 51 Pst -susceptible mutants (49.5%) had a deletion in the NLR 4DS-1 gene, of which 50 deletion events extended into RLK 4DS-2 but only 11 deletion events extended further to RLK 4DS-1 (Supplementary Data 4 ). However, no deletion only occurred in RLK 4DS-1 and/or RLK 4DS-2 . Among the remaining 52 non-deletion mutants, 18 Pst -susceptible mutants had at least one base change in the NLR 4DS-1 gene, and 16 of those mutations (89%) either caused an amino acid change or formed a premature stop codon (Supplementary Data 4 ). Seven amino acid variations were identified in the NLR 4DS-1 gene, including Gly117Asp, Val267Ile, Ser394Asn, Leu421Phe, Thr456Ile, Val482Ile, and Gln557Stop(*) (Supplementary Data 4 ). However, all 52 non-deletion mutants had no mutation in the coding region of RLK 4DS-2 . Thus, NLR 4DS-1 confers resistance to Pst in SW3 and Syn-SAU-93 and likely represents the YrAS2388R gene. Fig. 2 The YrAS2388 locus confers stripe rust resistance in wheat and barley. a Syn-SAU-93 and SW3 are two synthetic hexaploid wheat (SHW) lines that express the YrAS2388R gene. WT is the resistant wild-type control with necrotic lesions. L68 (G117D), L91 (V267I), F7 (S394N) and F43 (V482I) are susceptible mutants with sporulating Pst . Plant responses (MR = moderate resistance; R = resistant; S = susceptible) to Pst are indicated in parentheses. b The susceptible hexaploid wheat CB037 was transformed with the intact PC1104 (= F2-1). Transgenic T 3 wheat (all from the No. 5 and 10 T 2 subfamilies) was challenged with PSTv-239 at the adult plant stage. Under each picture, PCR results as positive (plus signs) or negative (minus signs) for DNA amplification (upper) and RNA expression (lower) of the three target genes: RLK 4DS-1 (left), RLK 4DS-2 (middle) and NLR 4DS-1 (right). RT-PCR is illustrated in Supplementary Fig. 4 . c The susceptible barley Golden Promise (GDP) was transformed with the intact PC1104 ( = F2-1). Transgenic T 1 barley seedlings were inoculated with race PSH-72 of Puccinia striiformis f. sp. hordei ( Psh ). Scale bar = 1 cm. Source data are provided as a Source Data file Full size image NLR 4DS-1 confers stripe rust resistance in wheat and barley We transformed wheat and barley with the fosmid PC1104 ( = F2-1; Supplementary Table 4 ), which has a 40-kb genomic fragment with NLR 4DS-1 , RLK 4DS-1 and RLK 4DS-2 . The spring wheat CB037 [34] was selected as the primary wheat recipient genotype because it is highly susceptible (IT scores = 7–9) to 11 Pst races, including PSTv-4, PSTv-14, PSTv-37, PSTv-39, PSTv-40, PSTv-47, PSTv-143, PSTv-221, PSTv-239, PSTv-306, and PSTv-353 (Supplementary Data 1 ). After bombarding 1,590 wheat immature embryos, we obtained 24 putative transgenic plants. NLR 4DS-1 , RLK 4DS-1 and RLK 4DS-2 were detected in four T 0 plants (No. 4, 5, 10, and 22), but only two plants (No. 5 and 10) were positive for the NLR 4DS-1 cDNA (Table 2 , Supplementary Fig. 4 ). For No. 5 and 10 transgenic plants, we selected 13 subfamilies that were homozygous resistant to PSTv-40 in the T 2 generation, and tested the T 3 plants against nine Pst races (PSTv-37, PSTv-39, PSTv-47, PSTv-143, PSTv-221, PSTv-239, PSTv-306, PSTv-352, and PSTv-353) and Pst spores from the field (Supplementary Data 1 ). The T 3 plants were resistant (IT scores = 0–4) to all Pst races at the seedling and adult-plant stages (Fig. 2b , Supplementary Fig. 5 , Supplementary Data 1 ). Table 2 Transgene expression and plant responses to Puccinia striiformis Full size table Barley cultivar Golden Promise is susceptible to race PSH-72 of the barley stripe rust pathogen, P. striiformis f. sp. hordei ( Psh ). After bombarding 2,200 barley immature embryos with PC1104, we obtained five putative transgenic lines. Only three T 1 families (No. 20, 34 and 35) segregated for their responses to PSH-72 (Table 2 , Fig. 2c ). T 1 plants with functional NLR 4DS-1 , RLK 4DS-1 and RLK 4DS-2 were resistant (IT scores = 1-5), while the ones lacking the three genes were susceptible (IT scores = 7–8). Therefore, the fosmid PC1104 confers stripe rust resistance in transgenic wheat and barley. Because PC1104 has NLR 4DS-1 , RLK 4DS-1 and RLK 4DS-2 genes, we cut PC1104 using a specific restriction enzyme (either Bsr GI, Kpn I, Not I, Xba I, or Kpn I + Xba I) to cleave/inactivate each of them, and then used the DNA fragments from each digestion to transform wheat separately (Supplementary Fig. 6 ). After bombarding 6,790 wheat immature embryos, we obtained 148 putative transgenic plants. Transgenic T 1 and T 2 plants were tested with Pst spores from the Parker Farm field (Moscow, ID, USA). Only transgenic plants that expressed NLR 4DS-1 were resistant to Pst (Table 2 , Supplementary Fig. 4 ). Therefore, NLR 4DS-1 represents a strong candidate for YrAS2388 (Table 2 ). The Pst -resistant NLR 4DS -1 has duplicated 3′UTRs (Fig. 1d ) in all Pst -resistant parents (CIae9, PI511383 and PI511384) and each 3′UTR is associated with multiple transcript variants: TV1 and TV2 with 3′UTR1, TV3 and TV4a (and 4b) with 3′UTR2 (Fig. 1e ). We overexpressed the Pst -resistant NLR 4DS-1 cDNA under the maize Ubi promoter (Supplementary Table 4 ). All 36 transgenic wheat and barley lines that expressed TV1 (or TV2) did not confer resistance to stripe rust (Table 2 ), suggesting that one cDNA isoform was insufficient to confer stripe rust resistance. For stripe rust resistance, the NLR 4DS-1 gene may require the activity of multiple cDNA isoforms and/or regulatory elements in the genomic sequence. Innate and external factors regulate NLR 4DS-1 expression In the Pst -resistant NLR 4DS -1 , the most abundant isoforms are TV1 (for a 1068-aa protein with complete 4HB, NB, and LRR domains) and TV4 (for a 471-aa protein with a complete 4HB and a partial NB domain) (Fig. 1e , Supplementary Fig. 7a ). The less abundant isoform TV2 might result from either a partial exon skipping from TV1 or the retention of an 833-bp cryptic intron in exon 5, which disrupts the NB and LRR domains. TV3 is also a less abundant isoform and is structurally similar to TV4, but retains the first 244 bp in the 833-bp cryptic intron, which only disrupts the LRR domain. In contrast, the Pst -susceptible NLR 4DS -1 either remained completely silent in PI486274 and PI560536 or produced only the TV1-type transcript in AL8/78 and AS87 (Supplementary Fig. 3b ). In Pst -resistant PI511383, TV1 to TV4 cDNAs were all expressed in the seedling and adult leaves (Supplementary Fig. 3c ). When exposed to alternating low (10 °C) and high (25 °C) temperatures, the high temperature upregulated TV2 and downregulated TV4 (Supplementary Fig. 3d ), which is correlated with increased Pst -resistance at elevated temperatures. In response to Pst race PSTv-306, the TV1 cDNA levels in the Pst -infected plants were comparable to those in the mock-inoculated control plants (Supplementary Fig. 3e ). In contrast, Pst infections upregulated TV2 at 2, 5, and 10 days post inoculation (dpi) but not at 3 dpi, downregulated TV3 at 3, 7, and 14 dpi, and downregulated TV4 at 3 dpi (Supplementary Fig. 3e ). Thus, both temperature and Pst infection regulate the transcription of NLR 4DS-1 . However, a change in the relative levels of either the individual four transcripts and/or the proteins or protein complexes may affect the induction of stripe rust resistance. Among the Pst -susceptible mutations of NLR 4DS -1 , Ser394Asn and Gln557Stop(*) only affect TV1 and Thr456Ile only affects TV4, which indicates that both TV1 and TV4 are essential for stripe rust resistance (Supplementary Data 4 ). Collectively, we hypothesize that TV1 plays a major role in the induction of stripe rust resistance, TV2 acts as a positive co-factor, and TV4 (or possibly TV3) act either as negative regulators when its expression is high or as positive regulators when its expression is low (Supplementary Fig. 8 ). Using a yeast two-hybrid system, we tested the interaction among the native (TV1, TV2, and TV4) and mutant (TV1 G117D , TV2 G117D and TV2 V267I ; Supplementary Data 4 , Supplementary Fig. 7a ) isoforms of the Pst -resistant NLR 4DS-1 . The NLR 4DS-1 isoforms, both native and mutant forms (NM forms) had no autoactivity. A strong interaction occurred amongst the TV2 proteins (NM forms; Supplementary Fig. 7b ). We observed a weak interaction between TV2 mutants and TV1 (NM forms), and between TV2 proteins (NM forms) and TV4. Apparently, TV2 can mediate protein interactions amongst multiple isoforms of NLR 4DS-1 . The Pst -resistant NLR 4DS - 1 occurs only in Aegilops tauschii The D genome of common wheat was derived from Ae. tauschii subsp. strangulata or tauschii [20] . The resistance allele of NLR 4DS-1 is present in 100% ( n = 37) and 19% ( n = 122) of the accessions of subsp. strangulata and tauschii tested, respectively (Supplementary Data 3 ). Similarly, the resistance allele of NLR 4DS-1 is present in 30% ( n = 23) of the Ae. tauschii accessions used as a parent in developing SHW lines (Supplementary Data 5 ). Surprisingly, the resistance allele is absent in all ( n = 461) of the common wheat lines tested (Supplementary Table 5 , Supplementary Data 6 ). The NLR 4DS-1 allele in Chinese Spring (CS) is nearly identical to the Pst -susceptible alleles from the subsp. tauschii accessions PI486274 and PI560636 (Supplementary Data 2 ). In addition, the resistant NLR 4DS-1 allele is also absent in all the tested T. monococcum subsp. aegilopoides ( n = 24), T. monococcum subsp. monococcum ( n = 24), T. turgidum subsp. dicoccoides ( n = 140), Ae. comosa ( n = 17), Ae. comosa var. subventricosa ( n = 6 ), Ae. longissimi ( n = 8), Ae. sharonensis ( n = 28), Dasypyrum villosum ( n = 10), and Hordeum vulgare subsp. spontaneum ( n = 5) (Supplementary Table 5 , Supplementary Data 6 ). The Pst -resistant NLR 4DS-1 may arise from paralogous genes All Pst -resistant NLR 4DS -1 genes contain two duplicated regions. The first region includes the 3′ end of exon 5, exons 6 and 7, and intron 7a; and the second region includes the pseudo-exon 5′, exons 6′ and 7′, and intron 7a′ (Fig. 1d, e , Supplementary Fig. 9a ). This duplication is not present either in Pst -susceptible NLR 4DS -1 alleles or in any NLR 4DS -1 -like genes. To examine the origin of the duplicated regions, we built separate phylogenetic trees for each of six selected fragments (exons 5, 6, 7, and 8; and introns 7a and 7b) of 7 to 15 NLR 4DS-1 homologues in Triticeae (Supplementary Fig. 9b ). The trees indicate that exons (5–8) and introns (7a and 7b) of the Pst -resistant NLR 4DS-1 are more related to those of the Pst -susceptible NLR 4DS-1 in CS (CS-4D:1821950..1825589); all the duplicated fragments (exons 5′ to 7′ and intron 7a′) are in separate clades. In addition, the duplicated 3′UTR1 and 3′UTR2 DNA of NLR 4DS-1 in PI511383 are only 87% identical in the conserved 373 bp (GenBank MK736661: 3735..4107 versus 6409..6781, counted forward from the start codon ATG). Thus, the Pst -resistant NLR 4DS-1 likely arose after a shuffling event between two paralogous genes. Specifically, the 3′UTR2 contains part of a 2668-bp insertion (within a 6-bp target site duplication = TACTGG) that occurred in intron 7 of the ancestral 3′UTR1 region. A similar 3′UTR duplication in the Pst -resistant NLR 4DS -1 gene is present in the synthetic wheat W7984 [35] . In the 2668-bp insertion, a 496-bp region (pseudo-exon exon 5′) is 90% identical to the ancestral exon 5. The insertion also has two miniature inverted-repeat transposable elements, which are frequently adjacent to transcriptionally active genes [36] . Likely, the 2668-bp fragment was derived from another, currently unidentified, NLR 4DS-1 homologue in Ae. tauschii . In Triticeae, there are multiple NLR 4DS-1 -like genes; three copies were identified in the YrAS2388 region (Supplementary Fig. 2 ). In common wheat CS, there are at least five transcriptionally active homologues of the NLR 4DS-1 gene (Supplementary Fig. 10 ). None of the NLR 4DS-1 -like homologues in CS has duplicated 3′UTRs. The Pst -susceptible NLR 4DS-1 homologues in CS share only 86%-94% identity with the Pst -resistant NLR 4DS-1 in PI511383 at the cDNA level. NLR 4DS-1 offers a toolbox for solving stripe rust problems We compared the stripe rust resistance in 81 SHW lines [33] and their original parents, including 30 SHW lines with the YrAS2388R gene (Supplementary Data 5 ). YrAS2388R confers a strong Pst resistance (IT scores = 1–3) in Ae. tauschii [22] . However, 27% of SHW wheat had significantly less resistance than the parental lines ( T. turgidum and/or Ae. tauschii ). In this study, SW3 has the Pst -resistant NLR 4DS-1 allele and shows the characteristic expression of alternatively spliced transcripts. However, SW3 was susceptible (IT scores = 7–9) to Pst in Moscow, ID, USA (Table 1 ), presumably because of a suppressor in its genetic background. Nonetheless, Ae. tauschii accessions with a strong Pst resistance frequently conferred moderate to high Pst resistance in a derived SHW wheat (Supplementary Data 5 ), indicating that Ae. tauschii is valuable for breeding resistant NLR 4DS-1 . For example, the SHW wheat Syn-SAU-S9 is based on Langdon/AS313//AS2399, in which the Ae. tauschii AS2399 is positive for the YrAS2388R gene [22] . Although Syn-SAU-S9 displayed only moderate resistance to Pst (IT scores = 4–5), we used Syn-SAU-S9 to transfer the YrAS2388R gene into common wheat. Three co-segregating markers were used for marker-assisted selection of YrAS2388R (Supplementary Fig. 11 , Supplementary Table 2 ). In 2015, we developed an elite line Shumai 1675, which is an F 6 line of Syn-SAU-S9/Chuan 07001//Shumai 969. Shumai 1675 is highly resistant to Pst in Sichuan, China. In 2017, Shumai 1675 outcompeted the check variety Mianmai 367 with an 11% increase in yield in the regional variety trials of the Sichuan province, China (Supplementary Table 6 ). YrAS2388R provides robust resistance in a wide spatial and temporal range, including China (current study), Canada [37] , Norway [25] , the United Kingdom [38] and the United States (TA2450 = CIae9, TA2452 = PI511384 [39] ; current study). However, YrAS2388R has had limited use probably for two reasons: it is absent in common wheat; and it can be suppressed in hexaploid wheat. In the present study, YrAS2388R , when separated from potential linkage drag, conferred strong stripe rust resistance in transgenic wheat and barley, indicating that YrAS2388R offers a practical solution for stripe rust resistance in Triticeae. The YrAS2388R gene-based markers (e.g. Xsdauw95 , Supplementary Fig. 11 ) can be used for marker-assisted selection. YrAS2388R is another example of a gene that was either not transferred or lost during domestication. Nevertheless, genes from both progenitors and distantly-related species of wheat can be used to enhance contemporary common wheat. Of the 81 permanently named Yr resistance genes, 21 were transferred from either related species or wild relatives of wheat, such as Yr5 from Triticum spelta , Yr15 and Yr36 from T. dicoccoides and Yr28 from Ae. tauschii [40] . However, alien genes can be accompanied by linkage drag [41] . For example, linked genes to Yr8 from Ae. comosa are associated with tall height and delayed maturity [42] . The Yr9 gene from the 1BL/1RS translocation improves grain yield but causes inferior quality [43] , which limits its use in wheat especially in the U.S. Pacific Northwest [44] . YrAS2388R could be transferred into wheat through a cisgenic approach. Thus, cisgenic YrAS2388R can provide an advantage to consumers in comparison to traditional breeding. YrAS2388R (or Pst -resistant NLR 4DS-1 ) is associated with duplicated 3′UTRs, which is an apparently rare phenomenon. The ancestral 3′UTR of NLR 4DS-1 adjoined the 3′-end of an unknown NLR 4DS-1 paralog, resulting in duplicated 3′UTRs in Pst -resistant NLR 4DS-1 . The 3′UTR is an important component of eukaryotic genes [45] . More than half of human genes use alternative polyadenylation to generate mRNAs that differ in the 3′UTR length but encode the same protein [46] . In contrast, there are few reports of genes with two separate 3′UTRs that cause a difference in the protein product. In wheat, the stripe rust resistance gene WKS1 generated six transcript variants, of which WKS1.1 differs from the others in the 3′UTRs [14] . Pst -resistant NLR 4DS-1 also shows alternative splicing (AS) in the NB-LRR region of the gene. AS is prevalent in eukaryotes [47] ; 95% of multi-exon genes in human [48] and 44% of multi-exon genes in Arabidopsis [49] display AS. In Arabidopsis, the bacterial-resistance gene RPS4 produces alternative transcripts in response to infection by pathogen Pseudomonas syringae pv. tomato [50] . Both environmental and developmental stimuli precisely regulate the abundance of functional mRNA isoforms [51] . Here, in keeping with resistance, expression of the NLR 4DS-1 isoforms also depends on pathogen infection and the temperature. Thus, abundance of NLR 4DS-1 isoforms appears to be a mechanism that wheat can use to robustly resist stripe rust pathogen invasion. The NLR 4DS-1 protein is a member of the CC-NB-LRR (CNL) proteins. The coiled-coil domain of the potato virus X resistance protein (Rx) actually forms a four-helix bundle (4HB) [52] . The N-terminal domain of NLR 4DS-1 is predicted to fold into four helixes, and it is also classified as an Rx-CC-like in the NCBI CDD (E = 9 × 10 −9 ) and Rx_N in the Pfam database (E = 6 × 10 −16 ). Although CNL genes are often race-specific and not durable [53] , some CNL genes such as the rice blast resistance gene Pigm R [54] have been durable. Here, we showed that YrAS2388R confers resistance to a broad array of Pst races and has been effective to all natural infections of Pst in China since 1995. As a typical NLR gene, we hypothesize that the NLR 4DS-1 proteins change their state via a competition model (Supplementary Fig. 8 ). The full-length TV1 protein plays a central role in signal transduction, but it requires other variant proteins (TV2 and TV4) for a proper conformation, which together form an active TV1 complex for defense signaling. Here, YrAS2388R was fully expressed without suppression in transgenic hexaploid wheat and in barley. In addition, we have produced Shumai 1675, which has YrAS2388R and is strongly resistant to Pst , suggesting that either YrAS2388R is not suppressed in Shumai 1675 or that YrAS2388R worked positively with other Yr genes to confer resistance to Pst . However, in the current study, the resistance levels of parental lines ( T. turgidum and/or Ae. tauschii ) were suppressed in nearly 27% of the SHW wheat lines. Yr28 , which is probably the same gene as YrAS2388 [22] , was effective in seedlings and adult plants of SHW Altar 84/ Ae. tauschii accession W-219 [24] . Here, we observed that YrAS2388R in SHW SW3 was suppressed, i.e., it was fully susceptible to natural Pst races at adult-plant stages in Moscow (ID, USA), probably because the suppressor responds more to the cooler night temperatures in this area. When YrAS2388R is suppressed in a specific hexaploid wheat such as SW3, Pst -resistance levels might be increased by disrupting the unknown suppressor, as was previously done by inactivating a suppressor of stem rust resistance [55] . In the case of wheat powdery mildew, pyramiding of closely related NLR genes can cause dominant-negative interactions and that lead to R gene suppression [56] . For example, the Pm8 resistance gene from rye was suppressed in wheat by a susceptible allele of the wheat ortholog Pm3 [57] . In the present study, the Pst -resistant NLR 4DS-1 in PI511383 shares 86–94% identity with cDNA from the transcriptionally active homologues in common wheat (Supplementary Fig. 10 ). Thus, YrAS2388R suppression might conceivably be caused by close homologues of NLR 4DS-1 that are present in Triticeae. To test this hypothesis, in the future, one could mutagenize a SW3 line, screen for truncation mutations in the NLR 4DS-1 homologues, and test whether the homologues’ mutations have any effect on stripe rust resistance. Regardless, because the transgene NLR 4DS-1 induces effective Pst resistance in hexaploid wheat, we predict that sustainable Pst resistance can be achieved with either a cisgenic strategy with Pst -resistant NLR 4DS-1 or a conventional strategy that combines both the incorporation of a Pst -resistant NLR 4DS-1 and either avoidance or inactivation of the apparently linked latent suppressor(s) from Ae. tauschii . Plant materials This study was performed on Aegilops tauschii , Hordeum vulgare , Triticum aestivum and synthetic hexaploid wheat (SHW [58] ) (Supplementary Table 7 ). Sources of accessions used for haplotype analysis are indicated in Supplementary Data 3 and 6 . To map YrAS2388 , we used six Ae. tauschii accessions (Supplementary Table 7 ), in which the Pst -resistant parents, CIae9, PI511383 and PI511384 (= AS2388), all have YrAS2388R [22] . We developed three F 2 populations (popA: PI511383/PI486274; popB: CIae9/PI560536; and popC: PI511384/AS87 [23] ). These populations were used for preliminary and fine mapping, and popC was also used to confirm the single Mendelian inheritance of YrAS2388 . In popA, we selected 11 F 2 plants that were heterozygous in the YrAS2388 region ( Xsdauw2 - Xsdauw36 ), and allowed them to self-pollinate to produce F 3 seeds. After screening 4,205 F 3 plants, we identified 467 plants with crossovers in the Xsdauw2 - Xsdauw36 interval, and used them to generate a high-density map. Stripe rust inoculum and infection assays Wheat stripe rust tests were conducted in four institutions: Shandong Agricultural University (SDAU), Tai’an, China; Sichuan Agricultural University (SCAU), Chengdu, China; Washington State University (WSU), Pullman, USA; and University of Idaho (UI), Moscow, USA. Avocet Susceptible (AvS), Huixianhong, Mingxian 169, and/or SY95-71 were used as susceptible checks and also planted surrounding the plots to increase and spread urediniospores for adequate and uniform rust levels for reliable screening. For winter-growth genotypes tested in greenhouses or growth chambers, seeds were vernalized in wet germination paper (Anchor Paper Co., Saint Paul, MN, USA) at 4 °C in darkness for 45 d; vernalized shoots were transplanted into soil in the greenhouse and maintained at 25 °C during the day and 15 °C at night with 16 h photoperiod. Infection types (IT) were recorded using a 0-9 scale [59] and the following categories: resistant (R, IT scores = 0–3), moderate reactions (M, IT scores = 4–6) that include moderate resistance (MR, IT scores = 4–5) and moderate susceptibility (MS, IT score = 6), and susceptible (S, IT scores = 7–9). IT scores were recorded 15–18 days post inoculation (dpi) when the uredinial pustules were clearly visible on susceptible plants. Responses of SHW and their parental lines to Pst are shown in Supplementary Data 5 . At SDAU, urediniospores were obtained from the Institute of Plant Protection, Chinese Academy of Agricultural Sciences, Beijing, China. Due to changes in race frequency and spore availability, different Pst races were used in different years (mixed spores of Chinese Pst races CYR29, CYR31, CYR32, CYR33, Su11 and/or Su14 during 2010 to 2012; CYR29 and CYR32 in 2013; and CYR29, CYR31, CYR32 and CYR33 in 2014–2016). Collectively, these races represent the predominant Pst races in China in different periods since the 1990’s. Field trials were performed to assess the responses to Pst in the parental lines, F 1 , F 2 and advanced progenies of popA and popB. At the seedling stage, an aqueous spore suspension was manually injected with a 2.5 ml syringe into leaf bundles and repeated after 10 days. For preliminary mapping, F 2 plants of popA and popB were evaluated in 2011, and the corresponding F 3 progeny were then tested in 2012. Critical recombinants of popA were evaluated in 2013-2016 (F 3 to F 6 generations, one generation per year), and the F 4 –F 6 generations were additionally tested in SCAU in 2014–2016. At SCAU, we primarily conducted the Pst test in Dujiangyan and Wenjiang, two experimental stations of the Triticeae Research Institute at SCAU. Urediniospores were obtained from the Research Institute of Plant Protection, Gansu Academy of Agricultural Sciences, Lanzhou, China. Using the mixture of Chinese Pst races CYR30, CYR31, CYR32, SY11-4, SY11-14, and HY46-8, we evaluated the Ae. tauschii germplasm in Dujiangyan for three growing seasons (2006–2009). In 2008–2009, we also tested synthetic wheat and their polyploid parents in Dujiangyan (Supplementary Data 5 ). Using a mixture of CYR30, CYR31, CYR32, CYR33, SY11-4 and HY46-8, we retested synthetic wheat and their parent lines in Wenjiang in 2011–2012 (Supplementary Data 5 ) [22] , and then retested five synthetic wheat and their parent lines in Wenjiang in 2016–2017 using a mixture of CYR32, CYR33, CYR34 (= Gui22-9), Gui22-14, and SY11-4 (Supplementary Data 5 ). To identify Pst -susceptible mutants, we screened the Syn-SAU-93 population in 2016–2018 and the SW3 population in 2017–2018 using urediniospores of similar races as 2016–2017. For popC, we assessed the parental lines, F 1 , F 2 and advanced progenies from 2010 to 2016. In 2011, F 2 plants were tested in Wenjiang, and the field plots were inoculated at 7 wk after planting with a mixture of CYR30, CYR31, CYR32, CYR33, SY11-4 and HY46-8. At WSU, urediniospores were produced by the USDA-ARS Wheat Unit at Pullman, WA, USA. The plants were initially grown in a greenhouse at 15 to 25 °C. At the two-leaf stage, we prepared a mixture of urediniospore and talc at 1:20 ratio (v vs. v), dusted it on plants, and then applied a water mist onto the plants. The inoculated plants were incubated in a dew chamber at 10 °C in the dark for 24 h, and then moved to growth chambers for either low or high temperature tests. The low temperature (LT) cycle had a 16-h photoperiod (6 a.m.–10 p.m.) with a diurnal temperature cycle of 4 °C at 2 am and a gradual increase to 20 °C at 2 pm followed by a gradual decrease to 4 °C at 2 am. The high temperature (HT) cycle had a 16-h photoperiod with a gradual temperature gradient from 10 °C at 2 a.m. to 30 °C at 2 p.m. and then back to 10 °C at 2 a.m.. At UI, urediniospores were produced by the USDA-ARS Wheat Unit at Pullman, WA, USA. Transgenic plants and wild-type controls were grown in chambers. At either the two-leaf stage for seedlings or at the 6-leaf stage for adults, plants were dust-inoculated using the urediniospore and talc mixture (1:20), maintained at 10 °C for 48 h in dark, and then maintained under a modified LT cycle (10 °C for 12 h with 8-h of darkness in the middle, 20 °C for 8 h in the middle of 16-h light, with a gradual transition from 10 to 20 °C within a 2-h light period and vice versa for a gradual transition from 20 to 10 °C) or under a modified HT cycle (15 °C for 12 h with 8-h darkness in the middle, 25 °C for 8 h in the middle of a 16-h light, with a gradual transition from 15 to 25 °C within a 2-h light period, and vice versa for a gradual transition from 25 to 15 °C). Bulked segregant analysis of the YrAS2388 gene Genomic DNA was extracted using the Sarkosyl method [17] . Infinium iSelect genotyping was assayed at the Genome Center (University of California, Davis, CA, USA). Normalized Cy3 and Cy5 fluorescence for each DNA sample was plotted with the GenomeStudio program (Illumina, Inc., San Diego, CA, USA), resulting in genotype clustering for each SNP marker [20] . We performed bulked segregant analysis (BSA) on four parents (CIae9, PI486274, PI511383 and PI560536) and 17 Pst -susceptible F 2 plants, ten from popA and seven from popB (Supplementary Table 1 ), using the wheat 10k iSelect array [29] . The Pst responses of the tested plants were obtained in the field in 2011. For SNP data, we sequentially eliminated: (1) those with missing data or that were being heterozygous in the parents, (2) those that were being polymorphic between the two resistant parents or between the two susceptible lines, (3) those that were identical among the four parents, and (4) those with four or more missing data points amongst 17 Pst -susceptible F 2 plants. We retained 3276 SNP loci for BSA analysis. Among Pst -susceptible F 2 plants with a clear genotype, the frequency of a homozygous “B” genotype (= susceptible phenotype) was calculated and sorted in descending order for each SNP. The top 20 SNPs were prioritized for further analysis. Preliminary and fine mapping of the YrAS2388 gene We targeted the AT4D3406 region (Supplementary Fig. 1a ) to develop PCR markers, which was facilitated by using the Ae. tauschii SNP map [29] , and the genome sequences of Ae. tauschii [30] , common wheat (IWGSC RefSeq v1.0 [60] ), synthetic wheat [35] and 20 fosmid clones of PI511383. Markers were primarily based on insertion-deletion polymorphisms (InDel), cleaved amplified polymorphic sequences (CAPS) and derived cleaved amplified polymorphic sequences (dCAPS [61] ). PCR primers, restriction enzymes and annealing temperatures are described in the Supplementary Table 2 . All other oligos used in the current study are documented in the Supplementary Table 8 . PCR products were separated in either 6% non-denaturing acrylamide or 2% agarose gels. The 4DS maps (Supplementary Fig. 1 ) were calculated using the maximum likelihood algorithm and the Kosambi function in JoinMap 4.0 (Kyazma B.V., Wageningen, Netherlands) and were assembled using MapChart v2.3 ( www.wur.nl/en/show/Mapchart.htm ). Construction and screening of the fosmid genomic library PI511383 leaf tissue was harvested from 4-week-old plants and stored at −80 °C. Megabase-size DNA was prepared by embedding nuclei in 0.5% low-melting agarose, followed by nuclear lysis in the presence of detergent and proteinase-K [62] . Sixty DNA plugs were transferred to individual 1.5-ml tubes with 200-μl TE buffer. DNA in agarose was sheared by 22 freeze-thaw cycles with incubation in liquid nitrogen for 20 s and then a 45 °C water bath for 3 min. The sheared DNA in a 33.5–63.5-kb range was purified from a gel, repaired using the DNA End-Repair enzyme, ligated into the pCC1FOS vector, and packed into the phage particles as instructed by the CopyControl™ Fosmid Library Production Kit (Epicentre Technologies Corp., Madison, WI, USA). Packaged fosmid clones were transformed into the EPI300-T1R competent cells, and the titer of the genomic library was calculated as indicated in the manual (Epicentre). On average, 1,000 or 2,000 clones per plate were obtained from a diluted solution after an 18 h to 24 h incubation at 37 °C. Colonies were recovered using a mix with 6 ml LB and 1.8 ml glycerol, divided into three aliquots (2 ml each, super colony pools), and stored at −80 °C. PCR screening was performed on each of 622 super colony pools, with 2-μl bacterium stock as template. We screened for markers Xsdau93 , Xsdau95 and O13 (PCR primers P160/P161) (Supplementary Tables 2 and 8 ). PCR amplification was performed as follows: 95 °C for 5 min, 32 cycles with 95 °C for 30 s, 58 °C for 30 s and 72 °C for 50 s, and a final extension at 72 °C for 10 min. PCR products were separated on a 1% agarose gel and visualized by ethidium bromide staining. For positive super colony pools, 25-μl glycerol stock was inoculated into 5-ml liquid LB supplemented with 12.5 μg chloramphenicol ml −1 (LB-C), and cultured on a 250 rpm shaker at 37 °C for 4 h. The culture was diluted in a 10-fold series (10 −1 to 10 −5 ) using liquid LB, and the serial dilutions (300 μl per level) were plated onto the LB-C agar. An ideal dilution yielded 4,000–5,000 clones per 15-cm-diameter plate, from which colonies were collected using the 384-pin replicator with four repeated contacts to collect more representative colonies. After the replicator was used to inoculate a 384-well plate with 50-μl liquid LB-C, the plate was incubated at 37 °C overnight. Each well was screened by PCR. For positive wells, 20-μl culture was enriched in 2-ml liquid LB-C, and grown in a 250 rpm shaker at 37 °C for 2 h. The end culture was diluted 10-fold (from 10 −1 to 10 −4 ) using liquid LB-C, and 100-μl culture was plated onto LB-C agar. An ideal dilution yielded 50–200 clones per 9-cm-diameter plate, from which a positive clone would be revealed among 24 clones. Mutagenesis and mutation screening Synthetic hexaploid wheat SW3 and Syn-SAU-93 were treated with 0.8% EMS (78 mM in water; Sigma-Aldrich Co., St. Louis, MO, USA). Briefly, lots of 400 seeds (M 0 ) were soaked in 100 ml EMS solution, treated on a shaker at 150 rpm. at 25 °C for 10 h, and washed with running water at room temperatures for 4 h. M 1 plants of SW3 were grown in a greenhouse in Taian, China. M 1 plants of Syn-SAU-93 were grown in the field in Chongzhou, China. To simplify the fieldwork, mutant seeds of SW3 and Syn-SAU-93 were bulk planted at M 2 to M 4 generations in Chongzhou and Wenjiang, respectively, and screened for Pst resistance using mixed urediniospores of races CYR30, CYR31, CYR32, CYR33, Gui22-1, SY11-4, and HY46-8 in 2016–2018. The Pst -susceptible mutants were screened for structural variations in the coding sequence of RLK 4DS-1 , RLK 4DS-2 , and NLR 4DS-1 . Plant DNA was prepared from the flag leaf using the Sarkosyl method [17] . Mutations of the candidate genes were identified using PCR-based DNA sequencing. For RLK 4DS-1 , we divided the 2570-bp fragment into two parts: (1) exons 1–3 between P162 and P163, and (2) exon 4 between P164 and P165. For RLK 4DS-2 , we examined a 1430-bp target region of the exon 3 between P167 and P168. For NLR 4DS-1 , we divided the 6072-bp fragment into five parts: (1) promoter and exons 1–3 between P169 and P170, (2) exon 4 between P171 and P172, (3) exon 5 between P173 and P174, (4) exon 5–6 between P175 and P176, and (5) the insertion region with 3′UTR2 between P177 and P178. PCR primers are described in the Supplementary Table 8 . A standard PCR reaction was performed with Taq polymerase (Promega, Madison, WI, USA). The PCR products were sequenced by the Sangon Biotech Company (Chengdu, Sichuan, China). Genetic transformation of wheat and barley The fosmid PC1104 (= F2-1; Supplementary Table 4 ) from PI511383 is about 47.7 kb (GenBank MK288012). PC1104 contains genomic copies of RLK 4DS-1 , RLK 4DS-2 and NLR 4DS-1 . Both intact and/or the restriction enzyme-cleaved PC1104 were used for wheat and barley transformation. For genetic transformations, we used four plasmids: (1) PC1104 for native expression of RLK 4DS-1 , RLK 4DS-2 , and NLR 4DS-1 , (2) Bsr GI, Not I, Xba I, Kpn I, or Xba I + Kpn I-cleaved PC1104 for native expression of RLK 4DS-1 , RLK 4DS-2 and NLR 4DS-1 , (3) PC1101 for overexpression of the NLR 4DS-1 TV1 cDNA, and (4) PC1102 for overexpression of the NLR 4DS-1 TV2 cDNA (Supplementary Table 4 ). To overexpress the candidate genes, we cloned the cDNA copies of NLR 4DS-1 TV1 cDNA with PCR primers P181/P182 and NLR 4DS-1 TV2 cDNA with PCR primers P181/P183. We then assembled two plant expression constructs: PC1101 ( Ubi::NLR 4DS-1 TV1-cDNA ) and PC1102 ( Ubi::NLR 4DS-1 TV2-cDNA ) (Supplementary Table 4 ). The fosmid PC1104 has no plant selection marker, and thus required co-transformation with PC174, which has the bialaphos ( BAR ) and hygromycin ( HYG ) selection markers both under the CaMV 35 S promoter (Supplementary Table 4 ). The other two plant expression constructs (PC1101 and PC1102) have both BAR and HYG selection markers on their T-DNA, and were used for direct transformation. Standard methods for biolistic bombardment and tissue culture of wheat were used [63] . Using an intact fosmid PC1104, we bombarded 1,590 immature embryos of CB037 and generated 24 putative transgenic plants. Using the cleaved fosmid PC1104 (Supplementary Fig. 6 ), we bombarded 5,790 immature embryos of CB037 and 2,013 immature embryos of Bobwhite, and generated 197 and 20 putative transgenic plants, respectively. Using the bombardment protocol for wheat [63] , we also transferred the intact fosmid PC1104 into barley Golden Promise, however the tissue culture and regeneration procedures were specific for barley [64] . We bombarded 2,200 immature embryos of Golden Promise and generated 300 putative transgenic plants. We also overexpressed the NLR 4DS-1 cDNA under the maize Ubi promoter in wheat and barley. For the NLR 4DS-1 TV1 cDNA (in PC1101), we bombarded 2,200 wheat immature embryos (Bobwhite or CB037), obtained 40 putative T 0 plants, and tested nine NLR 4DS-1 TV1 expressing T 1 families (seven of Bobwhite and two of CB037) for their response to PSTv-40. Using a standard Agrobacterium -mediated transformation [64] , we then infected 800 barley immature embryos (Golden Promise), obtained 15 putative transgenic T 0 plants, and tested four NLR 4DS-1 TV1 expressing T 1 families against PSH-72. For NLR 4DS-1 TV2 cDNA (PC1102), we bombarded 2,500 wheat immature embryos (Bobwhite), obtained 54 putative T 0 plants, and tested ten NLR 4DS-1 TV2 expressing T 1 families for their response to PSTv-40. We also then infected 800 barley immature embryos (Golden Promise), obtained 28 putative transgenic T 0 plants and tested 13 NLR 4DS-1 TV2 expressing T 1 families against PSH-72. Transgene integration was confirmed by a positive amplification of BAR with primers P184/P185, RLK 4DS-1 with primers P208/P209, RLK 4DS-2 with primers P203/P204 and NLR 4DS-1 with primers P213/P214 (or in the overexpression experiment with primers P186/P190). Transcription was assessed by RT-PCR with primers P208/P209 for RLK 4DS-1 , primers P187/P188 for RLK 4DS-2 , and primers P189/P190 for NLR 4DS-1 . ACTIN primers P191/P192 were used as an internal control for both wheat and barley. PCR primers are described in Supplementary Table 8 . Haplotype analysis Haplotype analysis was performed to understand the association of haplotypes and responses to Pst and the evolution of the YrAS2388 region. Haplotype markers (HTM) were specifically designed for RLK 4DS-1 , RLK 4DS-2 and NLR 4DS-1 . Their physical locations (in Supplementary Tables 3 and 5 , Supplementary Data 3 ) are counted from “A” in the start codon (ATG) in the genomic allele (GenBank accession number MK288012); for each marker, two periods separate the starting and ending nucleotides, and a minus sign indicates a backward count from “A” and a plus sign indicates a forward count from “A”. First, 159 Ae. tauschii accessions were genotyped in Sichuan, China using seven markers: HTM1a (= RLK 4DS-1 ), HTM2a (= RLK 4DS-2 ) and HTM3a to HTM3e (= NLR 4DS-1 ) (Supplementary Table 3 , Supplementary Data 3 ). Second, 874 Triticeae lines were genotyped in Shandong, China using four markers: HTM1b (= RLK 4DS-1 ), HTM2b (= RLK 4DS-2 ) and HTM3f to HTM3g (= NLR 4DS-1 ). PCR primers are described in Supplementary Table 2 . Markers used to genotype the Triticeae collection in Shandong were different from those used for genotyping the Ae. tauschii collection in Sichuan. Genotypes per gene per accession were not necessarily identical between the two tested collections. Thus, grouping of haplotypes should be considered separately for these two collections. Gene expression analysis RT-PCR was used to detect the expression of RLK1 4DS-1 , RLK1 4DS-2 , NLR 4DS-1 and ACTIN (internal control). Plants were maintained at 25 °C during the day and 15 °C at night with a 16 h photoperiod. Total RNA was extracted using TRIzol (Life Technologies, Grand Island, NY, USA). First strand cDNA was synthesized using the M-MLV Reverse Transcriptase (Invitrogen, Carlsbad, CA, USA). RT-PCR was conducted on the 2 nd -leaf of the juvenile (two-leaf stage) plants. Primers used were P193/P194 for RLK 4DS-1 , P195/P196 for RLK 4DS-2 , P197/P198 for NLR 4DS-1 and P191/P192 for ACTIN . Phusion High-Fidelity DNA Polymerase (Thermo Scientific, Wilmington, DE, USA) was used to perform the PCR reaction with 30 cycles for ACTIN , NLR 4DS-1 and RLK 4DS-1 and 38 cycles for RLK 4DS-2 . Quantitative real-time PCR (qRT-PCR) was used to measure four transcript variants of NLR 4DS-1 . qRT-PCR was conducted with SYBR Green reagents (Applied Biosystems, Foster City, CA, USA) on a StepOne Plus PCR System (Applied Biosystems). Specific PCR primers (Supplementary Table 8 ) were designed for four identified transcripts of the NLR 4DS-1 gene. Wheat ACTIN was used as an endogenous control [65] . Primers used were P215/P216 for NLR 4DS-1 TV1 , P217/P218 for NLR 4DS-1 TV2 , P219/P220 for NLR 4DS-1 TV3 , P221/P222 for NLR 4DS-1 TV4+ and P223/P224 for ACTIN . TV4 + also contains TV3, but TV3 only accounts for 2–5% of the total transcripts. The primer efficiencies were between 90% and 105%. Transcript levels were expressed as linearized fold- ACTIN levels calculated by the formula 2 ( ACTIN CT – TARGET CT) . Six biological replicates were used for each data point. Data were analyzed using the SAS program (v9.4). Sequence analysis Fosmid clones were extracted using QIAGEN Large Construct Kits (QIAGEN, Germantown, MD, USA). Library preparation, high-throughput sequencing and quality control were performed by the Berry Genomics Company (Beijing, China). In brief, DNA was fragmented, end-repaired, ligated to Illumina adaptors, and separated on a 2% agarose gel to select fragments about 400–500 bp [66] . Adaptor specific primers were used to amplify the ligation products. The final library was evaluated by qRT-PCR. PE reads (150 bp) were obtained using the Illumina HiSeq2500. Sequence reads of the vector pCC1FOS and the bacterial genome were masked by the crossmatch tool in the Phrap package [67] . A de novo assembly of each fosmid was done using either SPAdes 3.12 [ http://cab.spbu.ru/software/spades/ ] or ABySS 2.0.2 [ www.bcgsc.ca/platform/bioinfo/software/abyss/releases/2.0.2 ]. Orientation and order of small contigs was inferred using the reference sequences of W7984 [35] and AL8/78 [30] . Sequence gaps were filled by PCR clones and Sanger sequencing. Candidate genes were identified by searching Ensemble Plants [ http://plants.ensembl.org/index.html ] and the NCBI databases [ http://www.ncbi.nlm.nih.gov/ ]. The secondary and three-dimensional structures of the NLR 4DS-1 protein were predicted using PSIPRED [ http://bioinf.cs.ucl.ac.uk/psipred/ ] and Phyre2 [ http://www.sbg.bio.ic.ac.uk/phyre2/ ], respectively. Reporting summary Further information on research design is available in the Nature Research Reporting Summary linked to this article.